Ancient DNA reveals that bowhead whale lineages survived Late Pleistocene climate change and habitat shifts The climatic changes of the glacial cycles are thought to have been a major driver of population declines and species extinctions. However, studies to date have focused on terrestrial fauna and there is little understanding of how marine species responded to past climate change. Here we show that a true Arctic species, the bowhead whale ( Balaena mysticetus ), shifted its range and tracked its core suitable habitat northwards during the rapid climate change of the Pleistocene–Holocene transition. Late Pleistocene lineages survived into the Holocene and effective female population size increased rapidly, concurrent with a threefold increase in core suitable habitat. This study highlights that responses to climate change are likely to be species specific and difficult to predict. We estimate that the core suitable habitat of bowhead whales will be almost halved by the end of this century, potentially influencing future population dynamics. Climate change is a major selective force that can cause population declines or extinctions [1] , [2] , [3] , [4] . Darwin was one of the first to suggest that species could avoid extinction and remain in evolutionary stasis by tracking suitable habitat northwards and southwards during glacial cycles [5] . However, studies of ancient DNA (aDNA) have found that changes in numerous species’ distribution during the Late Pleistocene–Early Holocene transition were caused by the extinction of populations outside of isolated habitat refugia [1] , [6] , [7] . This is often associated with a loss of genetic diversity [7] , which is concerning because northwards habitat shifts are a common and global consequence of contemporary ongoing climate change [8] , [9] , [10] . However, most aDNA studies have been based on terrestrial species and little is known about the responses of marine species to climate change during the glacial cycles [11] . The bowhead whale is a true Arctic species that remains in polar waters throughout the year [12] . Like the polar bear, it is a sentinel species of the Arctic marine ecosystem due to its dependence on the sea ice [13] , [14] . Bowhead whales specialize in feeding on copepods and euphausiids, which are associated with primary production around the sea ice [12] , [13] , [14] . This ecological specialization and a long lifespan [15] make the bowhead whale a poor candidate for adapting to rapid climate change [13] , [14] ; thus the species is listed by the International Whaling Commission as being vulnerable to climate-induced disturbance [16] . However, bowhead whales are known to travel long distances within relatively short timescales [17] , [18] , which should enable the tracking of suitable habitat even in fast-changing environments. Radiocarbon dates of subfossil bowhead whales also suggest changes in presence and absence in the Canadian Arctic Archipelago that may be due to climate-induced range contractions and expansions during the Holocene [19] . Although bowhead whales are currently separated into five geographical stocks for management purposes, there is little genetic evidence of population structuring. Sea ice does, therefore, not appear to have been a barrier to movement between stocks, even those in different ocean basins, during warmer periods of the Holocene [20] , [21] . Previous aDNA studies have found that genetic diversity was maintained throughout the Holocene, despite bowheads being heavily exploited across their range by whalers [20] , [22] . Modelled projections based on Holocene data suggest that effective female population size increased in the Late Pleistocene [20] , [23] . However, it is not known whether these predicted changes in demography reflect changes in connectivity or overall population size [11] . Ancient DNA analysis of samples from the Late Pleistocene would allow the direct measurement of genetic parameters through this period of rapid climate change and potentially the inference of the underlying processes [11] . Here we present a multi-disciplinary study that utilizes aDNA and habitat suitability modelling to provide the first analysis of population dynamics of a marine species using a Late Pleistocene aDNA data set. Specifically, we use aDNA to verify the species identification of subfossils catalogued as bowhead whales based on morphology, but which could be right whales given their southerly distribution and the difficulty in distinguishing between the two taxa based on some morphological traits [24] . We model the distribution of the preferred habitat of the bowhead whale during the Late Pleistocene using paleoclimate data from the Last Glacial Maximum to investigate if the distribution of bowhead whale subfossils matched the predicted range. We test the hypothesis that, as with other Holarctic species, the bowhead whale would have suffered a demographic decline during the rapid climate change of the Late Pleistocene. We compare the genetic composition of Late Pleistocene samples south of 59°N with Early Holocene samples found North of 75°N to investigate whether these southern bowhead whales repopulated the Arctic following the retreat of the permanent sea ice. Finally, we use predicted climatic data to estimate the change in the distribution and extent of core suitable habitat for the bowhead whale by the end of this century. Species occurrence We carried out aDNA analysis on 44 subfossil bone samples that had been morphologically identified as possible bowhead whales. These samples originated from an area south of 59°N, over 1,000 km south of the current Arctic range of the bowhead whale [11] , [12] , [13] , [14] , [15] , [16] , [17] , [18] , [19] , [20] , [21] , [22] . We successfully genetically identified the species of 27 ancient samples, of which 15 were bowhead whales ( Supplementary Fig. S1 ). These southern bowhead whale samples were all radiocarbon dated to the Late Pleistocene ( Fig. 1 ). In contrast, nine of the younger, Holocene, samples from the same geographic range were genetically identified as the closely related North Atlantic right whale ( Eubalaena glacialis ) ( Fig. 1 , Supplementary Fig. S1 ), which occupies a more temperate climatic niche ( Fig. 2a ). This presence/pseudo-absence data strongly imply that the bowhead whale was replaced by its sister species, the right whale, at this latitude during the start of the Holocene. The North Atlantic right whale sequences were new haplotypes for this species, but clustered with previously sequenced haplotypes from the western North Atlantic stock, suggesting there may have been low population structuring between the eastern and western North Atlantic ( Supplementary Fig. S2 ). 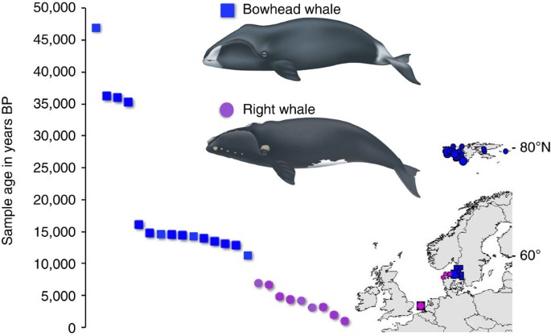Figure 1: Changes in species occurrence during the Pleistocene–Holocene transition. Ancient DNA analysis of radiocarbon-dated balaenid subfossils identified the occurrence of a true Arctic species, the bowhead whale, south of 59°N during the Pleistocene, which is then replaced by the right whale during the Holocene. Insert shows a map of the study area and locations of the samples used in this study: Late Pleistocene bowhead whale subfossil samples (blue squares); Early Holocene bowhead whale subfossil samples22(blue circles); and Early Holocene right whale subfossils (purple circles). Figure 1: Changes in species occurrence during the Pleistocene–Holocene transition. Ancient DNA analysis of radiocarbon-dated balaenid subfossils identified the occurrence of a true Arctic species, the bowhead whale, south of 59°N during the Pleistocene, which is then replaced by the right whale during the Holocene. Insert shows a map of the study area and locations of the samples used in this study: Late Pleistocene bowhead whale subfossil samples (blue squares); Early Holocene bowhead whale subfossil samples [22] (blue circles); and Early Holocene right whale subfossils (purple circles). 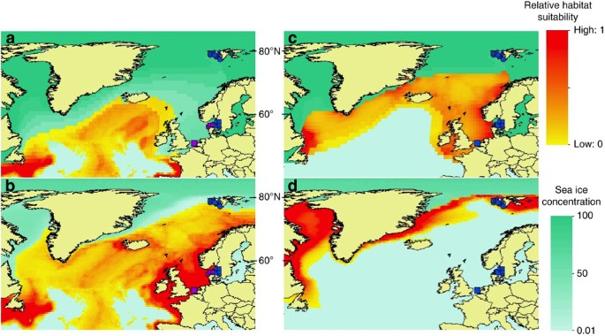Figure 2: Modelled predictions of suitable habitat. Predicted suitable habitat for right whales during (a) the Last Glacial Maximum and (b) the Holocene; and for bowhead whales during (c) the Last Glacial Maximum and (d) the Holocene. Red areas correspond to core suitable habitat as defined in theSupplementary Methods. Locations of the samples used in this study are marked as: Late Pleistocene bowhead whale subfossil samples (blue squares); Early Holocene bowhead whale subfossil samples22(blue circles); and Early Holocene right whale subfossils (purple squares). Full size image Figure 2: Modelled predictions of suitable habitat. Predicted suitable habitat for right whales during ( a ) the Last Glacial Maximum and ( b ) the Holocene; and for bowhead whales during ( c ) the Last Glacial Maximum and ( d ) the Holocene. Red areas correspond to core suitable habitat as defined in the Supplementary Methods . Locations of the samples used in this study are marked as: Late Pleistocene bowhead whale subfossil samples (blue squares); Early Holocene bowhead whale subfossil samples [22] (blue circles); and Early Holocene right whale subfossils (purple squares). Full size image Habitat modelling The distribution of the Late Pleistocene bowhead whale subfossils overlapped with areas of core suitable habitat, which were predicted using AquaMaps [25] based on climate data from the Last Glacial Maximum (LGM; Fig. 2c ). During this period, much of the bowhead whale’s current range would have been inaccessible due to the extent of the permanent sea ice ( Fig. 2c ), and so could not have supported a refugial population. The occurrence of early Holocene subfossils in the high Arctic [20] , [22] also overlapped with the predicted geographic range of suitable habitat for bowhead whales during the Holocene ( Fig. 2d ). The most southerly bowhead whale samples, found off the coast of the Netherlands, were also the oldest (>30,000 years BP). No bowhead whales were dated to the LGM, during which most of the North Sea would have been dry land [26] . The younger bowhead whale samples (10,000–14,000 years BP) were all found around northern Denmark and southern Sweden ( Supplementary Table S1 ). Population structure and dynamics We compared the Late Pleistocene samples with two data sets from the Arctic dated to the Early Holocene [19] , [22] to determine whether the southern lineages repopulated the Arctic following the rapid climate change that occurred between these sampling periods. The first comparison with 34 samples from Svalbard [22] , which is almost directly north of the locations of our Late Pleistocene subfossils, revealed four shared haplotypes and no significant differentiation (Φ ST =0.008, P =0.252) between the two time periods ( Fig. 3 ). The second comparison with a data set of Early Holocene subfossils from the Central Canadian Arctic [20] identified three shared haplotypes and no significant differentiation (Φ ST =0.003, P =0.473) between the two time periods. 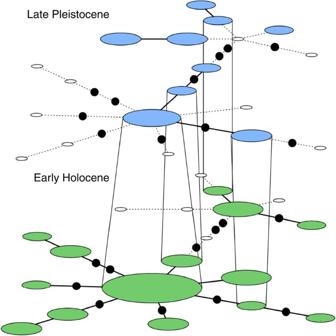Figure 3: Survival of bowhead whale lineages during the Pleistocene–Holocene transition. A haplotype network illustrates the survival of the lineages of bowhead whales found south of 59°N during the Late Pleistocene through to the early Holocene, when bowhead whales were found in their current Arctic range. The haplotype network is stratified into two time periods: the top network (blue) indicates data from the Late Pleistocene and the lower network (green) indicates data from the Early Holocene22. Vertical lines link haplotypes found in both time periods. Circles are proportional to haplotype frequency in that time period. White circles indicate haplotypes found in one time period, but not the other; black circles indicate inferred haplotypes. Figure 3: Survival of bowhead whale lineages during the Pleistocene–Holocene transition. A haplotype network illustrates the survival of the lineages of bowhead whales found south of 59°N during the Late Pleistocene through to the early Holocene, when bowhead whales were found in their current Arctic range. The haplotype network is stratified into two time periods: the top network (blue) indicates data from the Late Pleistocene and the lower network (green) indicates data from the Early Holocene [22] . Vertical lines link haplotypes found in both time periods. Circles are proportional to haplotype frequency in that time period. White circles indicate haplotypes found in one time period, but not the other; black circles indicate inferred haplotypes. Full size image The Late Pleistocene bowhead whale sequences were compared with a data set of 99 Holocene bowhead whale sequences from subfossils collected from Svalbard in the Arctic [22] . The skyline plot estimated from these sequences ( Fig. 4 ) did not detect any loss of genetic diversity due to a founder effect in early Holocene Arctic bowhead whales. This is contrary to predictions arising from the leading-edge model of post-glacial expansion [4] , [27] . Conversely, using coalescent-based estimation of changes in effective female population size through time, based on a data set of 114 radiocarbon-dated mitochondrial DNA sequences of bowhead whales spanning 50,000 years, we detect an approximately sixfold increase during the Pleistocene–Holocene transition ( Fig. 4 ). Therefore, bowhead whales are an unusual case study, as most terrestrial Holarctic mammals that have been studied using aDNA went through demographic declines or went extinct at the end of the Pleistocene [1] , [3] , [7] . The area of predicted suitable core habitat of bowhead whales tripled during the rapid climate transition between the Late Pleistocene and Early Holocene ( Fig. 2c ), concurrent with the detected increase in effective population size ( Fig. 4 ). 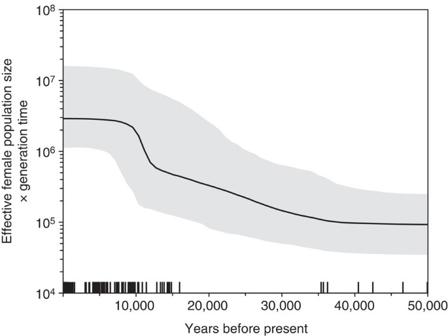Figure 4: Skyline plot showing temporal changes in genetic diversity in bowhead whales. Thexaxis is in calendar years; theyaxis is the product of effective population size and generation time (Neτ). The temporal span of the radiocarbon-dated samples used in this analysis is shown as vertical lines below thexaxis; each line represents one dated individual. Figure 4: Skyline plot showing temporal changes in genetic diversity in bowhead whales. The x axis is in calendar years; the y axis is the product of effective population size and generation time ( N e τ). The temporal span of the radiocarbon-dated samples used in this analysis is shown as vertical lines below the x axis; each line represents one dated individual. Full size image Forecasted change in core suitable habitat There has been a significant linear warming of the upper 300 m of the world’s oceans in recent decades [28] , [29] . This increase is almost twice as large in Arctic waters due to Arctic amplification, a feedback mechanism whereby the loss of sea ice increases the rate of temperature rise, which in turn increases the rate of loss of sea ice [29] . As a consequence, it is expected that sea ice will further and rapidly diminish from Arctic waters in the next few decades. Modelling future habitat distribution using AquaMaps [25] , we predict a loss of almost 50% of core suitable habitat for bowhead whales by the year 2100 ( Fig. 5 ). 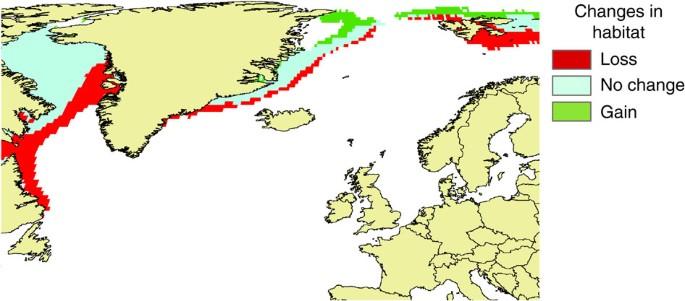Figure 5: Changes in predicted bowhead whale core suitable habitat by the year 2100. Red areas are predicted to be lost by 2100, green areas are predicted to become core suitable habitat by the year 2100 and turquoise areas are not expected to change in habitat suitability. Figure 5: Changes in predicted bowhead whale core suitable habitat by the year 2100. Red areas are predicted to be lost by 2100, green areas are predicted to become core suitable habitat by the year 2100 and turquoise areas are not expected to change in habitat suitability. Full size image Our analysis of the population dynamics of bowhead whales has documented the survival of lineages through the Pleistocene–Holocene transition, with evidence of an increase in effective female population size concurrent with a shift in geographic distribution. This is in contrast with many terrestrial Holarctic mammals, which suffered population declines or went extinct altogether during the Late Pleistocene [1] , [3] , [4] , [6] , [7] , [26] , [30] . Cold-adapted Arctic species are thought to have been in a contraction phase and living in refugia during inter-glacials such as the Holocene [1] , [4] , [6] . However, our findings of increases in both core suitable habitat and effective female population size during the Holocene suggest that bowhead whales do not follow this pattern, providing further evidence that responses to climate change are likely to vary among species [3] . The ability to adapt to climate-induced shifts in habitat distribution may therefore sometimes depend on changes in the amount, rather than distribution, of suitable habitat available for a species. Additionally, the lower energetic cost of movement may make habitat tracking more feasible for marine than terrestrial species [31] . It is also important to consider that population structuring of bowhead whales and other Arctic marine mammals is likely to have changed during the climatic shifts of the Late Pleistocene–Early Holocene transition [11] . Bowhead whales in the Atlantic and Pacific were probably isolated from each other by the ice sheets during the Late Pleistocene [32] . In contrast, the Northwest Passage was thought to be open to bowhead whales at the start of the Holocene, with the greatest frequency of bowhead subfossils in the Canadian Arctic Archipelago occurring between 11,000 and 9,000 years ago [32] . Previous aDNA studies of the bowhead whale showed that there has been connectivity between the Bering-Chukchi-Beaufort Seas, the Central Canadian Arctic and Svalbard-Barents Sea stocks during periods of the Holocene [20] , [21] , [22] . Therefore, the increase detected in effective female population size at the end of the Pleistocene may be linked to habitat increase, but may also reflect an increase in connectivity between the Atlantic and the Pacific. The lack of genetic differentiation between the Late Pleistocene and Early Holocene samples suggests we were unable to detect potential recent migrants from the Pacific. Given the substitution rate of 2 × 10 −7 substitutions per site per year [33] and a separation of stocks lasting approximately 10,000 years during the LGM, we would not expect sufficient sequence divergence to be generated between Pacific and Atlantic bowhead whales to be able to distinguish between them. Given the lack of phylogeographic structure in this species, we are unable to conclusively determine the relative contribution of the Late Pleistocene samples included in this study to the repopulation of the northern habitats. However, we can make some inferences. Previous studies suggested that the Arctic habitat of the bowhead whale was unavailable to them while it was glaciated during the Last Glacial Maximum. From 99 samples found around Svalbard, three were dated to 40,000–51,000 years BP, the remainder were dated to 11,000 years BP or younger [22] . Furthermore, all of the >400 bowhead whale remains found in the Canadian Arctic were radiocarbon dated to 10,500 years BP or younger [19] . Therefore, it seems unlikely that the bowhead whales that contributed to the Holocene populations survived in northern refugial populations during the Late Pleistocene. Following deglaciation, the waters around Svalbard would have been reoccupied by bowhead whales from either more southerly waters in the Atlantic or from the Pacific. Therefore, some northerly movement and large-scale migrations must have taken place. A genetic study of bowhead whale subfossils from along the coast of Norway as the sea ice retreated would shed further light on how bowhead whale lineages tracked the retreating ice sheets. The potential relationship between the extent of core suitable habitat and effective female population size has implications for bowhead whale conservation, given our prediction of a 50% decrease in core suitable habitat by the year 2100. The extreme depletion of the North Atlantic bowhead population through whaling over the past three centuries may mean that population growth is unlikely to be constrained by habitat availability in the immediate future. Nevertheless, if population responses to past climatic change are indicative of future responses, cumulative impacts related to climate change and the associated habitat loss may eventually limit the carrying capacity of bowhead whale populations. Furthermore, if populations respond to ongoing directional climate change by shifting their distribution northwards to track the retreating sea ice, then the endangered Okhotsk Sea population may become increasingly isolated and vulnerable [11] . Therefore, as with other Arctic species dependent on sea ice such as polar bears [34] , measures to mitigate climate change and sea ice reduction are needed if bowhead whales are to be effectively conserved. DNA extraction and amplification Subfossil baleen whale samples were sampled following the protocol outlined in McLeod et al . [20] , from collections held at the Zoological Museum, University of Copenhagen; Natural History Museum, Rotterdam; Gothenburg Museum of Natural History; Gothenburg Stadsmuseum; Vendsyssel Historical Museum; Museumcenter, Hanstholm; and Natural History Museum of Aarhus. Previous genetic studies have shown that bowhead whale B. mysticetus and right whale E. glacialis skeletal remains cannot always be reliably distinguished based on morphology [24] . Given that many of our samples were from vertebrae, from which curators suggested they could not conclusively distinguish among taxa, species identification was molecularly determined using aDNA protocols. All laboratory work on unamplified DNA was carried out in a designated clean lab, set up specifically for aDNA analyses. Blank DNA extractions and PCRs were incorporated to monitor for contamination. No modern whale DNA was present in the same building. Workflow conformed to aDNA protocols, that is, individuals did not return to the clean lab on the same day following working in post-PCR areas. All post-PCR laboratory work on amplified DNA was conducted in a separate laboratory facility. DNA was extracted and purified from approximately 0.01–0.19 g (sample dependent) of powdered bone. Blank extractions were included every five samples to monitor for contamination. PCR amplification of 219 bp of the hypervariable region of the mtDNA d-loop was conducted using primer pairs fwd1 5′-TTCACTACGGGAAGTTAAAGCTCG-3′ and rev1 5′-GGAGCGGCCATAGGATTCAGTTG-3′; fwd2 5′-CCGCTCCATTAGATCACGAG-3′ and rev2 5′-CTGAAGTAAGAACCAGATGTCT-3′; fwd3 5′-CAGGGATCCCTCTTCTCGCA-3′ and rev3 5′-CCATCGWGATGTCTTATTTAAGRGGAA-3′ resulting in two non-contiguous fragments corresponding to positions 15,676–15,753 and 15,791–15,927 of the bowhead whale mitochondrial genome. Each 25 μl PCR contained 5 μl of extracted DNA, 1 × buffer, 2.5 mM MgCl 2 , 1 mM of each primer, 1 mM mixed dNTPs and 0.2 μl AmpliTaq Gold enzyme (Applied Biosystems). PCR amplifications were performed using an MJ Thermocycler with a 4 min activation step at 95 °C, followed by 50 cycles of 95 °C for 20 s, 54 °C for 30 s, 72 °C for 20 s, followed by a final extension period of 72 °C for 7 min. PCR negative controls without DNA were included for every three samples amplified to monitor for contamination during the PCR set up. To guard against the incorporation of erroneous data derived from DNA damage or contamination, the PCR amplification and sequencing process was replicated twice for each sample. The amplified PCR products were purified using a Qiagen MinElute PCR purification kit. The product was cloned with the Invitrogen TA cloning system, and 16 colonies per sample were sequenced with the commercial facility offered by Macrogen (Seoul, Korea). DNA data analysis Species identification was determined by comparing with sequences in GenBank using the BLAST algorithm (see Supplementary Table S1 ) and by building a maximum likelihood phylogenetic tree performed using PHYML 3.0 (ref. 35 ). The HKY model of nucleotide substitution [36] was selected based on the Bayesian information criterion using Modelgenerator [37] . The transition/transversion ratio, the proportion of invariable sites, the gamma distribution and the starting tree, estimated using a BIONJ algorithm [38] , were also estimated by PHYML 3.0. The reliability of the optimized tree was estimated using the approximate Likelihood Ratio Test method with Shimodaira-Hasegawa-like support [39] ( Supplementary Fig. S1 ). Sequences identified as right whale were aligned by eye with previously published right whales DNA sequences from GenBank, and these were built into a phylogenetic tree as above ( Supplementary Fig. S2 ). Sequences identified as bowhead whale were aligned by eye with previously published bowhead whales DNA sequences from samples from Svalbard dated to the early Holocene (11,000–8,500 BP) [22] and visualized as a heterochronous parsimony network using TempNet (ref. 40 ). To estimate population history, a Bayesian skyline analysis was conducted using the phylogenetic software BEAST v1.7.2 (ref. 41 ). The HKY+G model of nucleotide substitution [36] was selected based on the Bayesian information criterion using Modelgenerator [37] , with rate heterogeneity among sites modelled using a discrete gamma distribution with six rate categories. Population history was inferred using the Bayesian skyline plot with six groups of coalescent intervals. Estimates of the substitution rate and coalescence times were calibrated using the radiocarbon ages of the samples. To evaluate whether these sampling times presented sufficient temporal information for calibration, we analysed ten replicate data sets in which the sampling times were randomized among sequences [42] . All ten replicate data sets yielded rate estimates that did not overlap with the mean rate estimated from the original data set, suggesting that the sampling times provide sufficient calibrating information. Posterior distributions of parameters, including the tree, were estimated using Markov chain Monte Carlo sampling. Samples were drawn every 5,000 steps over a total of 50,000,000 steps, with the first 10% of samples discarded as burn-in. Convergence to the stationary distribution and sufficient sampling were checked using Tracer v1.5 ( http://tree.bio.ed.ac.uk/software/tracer ) [41] . We repeated the analysis using an age-dependent model of post-mortem damage [43] , but a Bayes factor analysis yielded decisive support for the original model (without post-mortem damage). Furthermore, the 95% credibility interval of the damage parameter included a value of zero, suggesting that there is no evidence of appreciable post-mortem damage in the sequence data. Power analyses to see if the data could be used to compare nucleotide diversity between time periods were conducted following McLeod et al . [20] , but power was low as previously found by McLeod et al . [20] and this comparison is not included here. New mitochondrial sequence data have been deposited at GenBank ( Supplementary Table S1 ). Radiocarbon dating Several samples had been radiocarbon dated by previous studies [44] . The remainder were AMS dated at the 14 CHRONO Centre, Queens University Belfast. C:N ratio was between 3.2 and 3.4, indicating acceptable preservation of collagen [45] . The results in Supplementary Table S2 were calibrated using the INTCAL09 Marine modelled curve [46] . Accounting for a reliable reservoir offset is difficult, as the reservoir may vary through time in single locations and the mammals themselves are migratory species and their protein intake varies, and probably crosses different reservoirs [47] . For this reason we have corrected the radiocarbon dates using a delta-R value of 0 and estimated an uncertainty of 40 years. For radiocarbon determinations of ~10 ka BP or older this uncertainty makes little overall difference, but of course it can be manifestly more significant for younger measurements. However, it does not alter the conclusions of this paper. Habitat suitability modelling We used the AquaMaps approach ( http://www.aquamaps.org ) to species distribution modelling for mapping current, potential Pleistocene and future bowhead and North Atlantic right whale ranges [48] . AquaMaps is a bioclimatic envelope model that combines existing point occurrence data with available expert knowledge on species occurrence in environmental and geographic space to generate large-scale predictions of the relative occurrence of marine species. In this context, habitat usage of species can be described based on a predefined set of environmental parameters including depth, temperature, salinity, primary production and sea ice concentration, which is subsequently projected into geographic space in a global grid of 0.5 degree latitude by 0.5 degree longitude cells. As an environmental niche model, AquaMaps was developed specifically to deal with non-representative sampling of marine species ranges, but also to address the prevailing overall paucity of available point occurrence records by incorporating expert knowledge on species habitat usage. For bowhead whales specifically, there is currently only a single record available through OBIS ( http://www.iobis.org ). Similarly, bowhead whale records accessible through GBIF that can be used as input data of species distribution models are almost equally rare: only 11 out of >1,000 bowhead whale specimen records accessible through GBIF ( http://www.gbif.org ) are identified as geo-referenced observations of live animals (that is, sightings). However, all of these records are clustered along the US Alaskan coastline in the Beaufort Sea, thus making it problematic to directly base predictions of species occurrence in the North Atlantic on these data alone using standard presence-only species distribution modelling (SDM) approaches such as Maxent [49] . Using AquaMaps allowed the verification of environmental envelope settings, calculated from available point data, and the resulting extrapolated species occurrence in the North Atlantic during an iterative review process involving several species experts. Resulting model outputs are highly consistent with available other range maps such as NOAA ( http://www.nmfs.noaa.gov/pr/pdfs/rangemaps/bowheadwhale.pdf ) and the IUCN ( http://maps.iucnredlist.org/map.html?id=2467 ) and checked by colleagues familiar with the distribution of this species. Similarly, use of expert knowledge allowed modelling of the pre-exploitation range of North Atlantic right whales, including the Northeastern Atlantic where there are almost no point locality data, as whaling extirpated the species several centuries ago in these waters. For the purpose of this study, we used a slightly modified version of AquaMaps default, expert-reviewed, envelope settings for both, bowhead and North Atlantic right whales. Specifically we excluded primary production from the model, as there are no data for Pleistocene conditions including this parameter ( Supplementary Table S3 ). Comparisons of Fig. 2d with AquaMaps predictions for bowhead whales, which included this parameter ( http://www.aquamaps.org/preMap2.php?cache=1&SpecID=ITS-180533 , reviewed version 2012-07-13) and outputs from a similar model using distance from the ice edge as an input parameter ( [50] , p. 164) indicated that model outputs are fairly robust to these changes, resulting in just some localized changes in the relative suitability of habitat. We projected predictions of relative probability of whale occurrence based on local conditions into geographic space using environmental data for different time periods, assuming no changes in species-specific habitat usage over time. As the climate has been relatively stable throughout the Holocene, with variability being small compared with the difference between glacial cycles [51] , current environmental conditions were assumed to be representative of conditions throughout the Holocene. Current distribution was based on the compiled standard AquaMaps environmental data, as described by the meta-data available at http://www.aquamaps.org/download/main.php . Pleistocene environmental conditions reconstructed for the last glacial maximum (~20,000 calendar years before presence) as part of the GLAMAP project [52] were used in the hind-casting scenario. We computed mean annual environmental conditions during the Pleistocene based on the available interpolated winter and summer predictions for sea surface temperature and salinity deduced from sediment core data [52] . As an approximation for mean annual sea ice concentration required as input by the AquaMaps model, we used the mean proportion of time a given cell had been defined to be covered by ice in the GLAMAP data set [52] . Future annual average environmental conditions for the 2091–2100 decade were based on the Special Report on Emissions A2 climate change scenario [53] . Applying a presence threshold of 0.6, as indicated by recent validation analysis [54] , we predict a loss of 47% of core suitable habitat (throughout the whole range) for bowhead whales by the year 2100 and an increase in core suitable habitat of 69% after the end of the Pleistocene. Accession codes: The bowhead whale mitochondrial genome sequences were deposited in GenBank under the accession codes: AJ554051.1 and KC573762—KC573781 How to cite this article: Foote, A.D. et al . Ancient DNA reveals that bowhead whale lineages survived Late Pleistocene climate change and habitat shifts. Nat. Commun. 4:1677 doi: 10.1038/ncomms2714 (2013).